Allelic variation at a single gene increases food value in a drought-tolerant staple cereal The production of adequate agricultural outputs to support the growing human population places great demands on agriculture, especially in light of ever-greater restrictions on input resources. Sorghum is a drought-adapted cereal capable of reliable production where other cereals fail, and thus represents a good candidate to address food security as agricultural inputs of water and arable land grow scarce. A long-standing issue with sorghum grain is that it has an inherently lower digestibility. Here we show that a low-frequency allele type in the starch metabolic gene, pullulanase, is associated with increased digestibility, regardless of genotypic background. We also provide evidence that the beneficial allele type is not associated with deleterious pleiotropic effects in the modern field environment. We argue that increasing the digestibility of an adapted crop is a viable way forward towards addressing food security while maximizing water and land-use efficiency. Food security is a key challenge facing humanity, given the exponential population growth and climate change [1] , [2] . Increasing production without agricultural expansion remains at the core of proposed solutions to ensure food security while minimizing environmental impact [3] . Little attention, however, has been given to improving the intrinsic, usable, caloric value of staple foods as a way to tackle food insecurity. This is particularly important in regions such as Africa where malnutrition is rife because of economic, climatic, environmental and social instability [4] , [5] . Sorghum ( Sorghum bicolor (L.) Moench), a cereal domesticated in Africa, is central to addressing the challenges of securing a food supply while being pre-adapted to climate scenarios that have been forecasted [5] , [6] . Sorghum is drought tolerant, can grow in regions otherwise unfit for other cereals, but unfortunately suffers from lower digestibility compared with other cereals [7] , [8] . Aside from being a crop that is well adapted to address food insecurity, sorghum has garnered attention as a biofuel feedstock with efficiency advantages over maize [9] . Understanding and improving starch metabolism and accumulation is of central importance to cereal genetics and breeding, as starch constitutes the majority of calories in grain [10] , [11] . Mutations in genes encoding starch metabolic enzymes have been known for some time to alter the structure, properties and digestibility of starch in major cereals [11] , [12] , [13] , [14] . These mutations in starch-biosynthesis genes, however, can have pleiotropic effects on other important agronomic traits including yield, limiting their usefulness to modern breeding programs [15] . It is therefore important to find mutations in starch-biosynthesis genes that are unlikely to have pleiotropic effects on plant growth and yield, in order to improve the digestibility and caloric value of cereal crops. Initially, we examined starch metabolic genes (starch branching enzymes, starch synthases and starch de-branching enzymes) across diverse genotypes in an effort to investigate whether non-synonymous mutations correlated with grain quality phenotypes. Pullulanase (EC 3.2.1.41) is a starch metabolic enzyme and is encoded by loci that are widely conserved across plants and bacteria [16] . In Viridiplantae with searchable, publically available sequence data, pullulanase is a single to low-copy gene. Plant pullulanase preferentially removes short chain maltodextrins from branched polysaccharides through α 1→6 bond cleavage [17] . Knockouts of maize and rice pullulanases result in the loss of pullulanase activity (PA) without readily detectible phenotypic changes in plant growth or grain phenotypes [16] , [18] . Pullulanase function overlaps partially with the de-branching isoamylases and it has been reasoned that pullulanase knockouts are still viable because of activity of the isoamylases [16] , [19] . Cereal pullulanase function may therefore be dispensable for normal plant growth, despite being a part of the primary starch metabolic machinery. It remains to be determined, however, whether changes in PA influences digestibility in major cereal crops, thus we attempted to find any interactions between digestibility and variation at the pullulanase locus in sorghum. Here we test this hypothesis by investigating whether polymorphisms in pullulanase can increase starch digestibility without pronounced pleiotropic effects on plant growth and yield in sorghum. The motive was to search for non-silent polymorphisms that may better define starch metabolic gene function in sorghum, particularly through missense mutations in diverse landraces. In doing so, we discovered a pullulanase allele type that positively has an impact on the starch digestibility of sorghum grain, a solution to the long-standing issue with this important crop [8] , [20] . We show that a naturally occurring allele type of the starch metabolic gene, pullulanase, confers higher in vitro digestibility ( iv D) and enzymatic activity, but surprisingly occurs at low frequency. At high frequency, we find a pullulanase allele type associated with dramatically reduced digestibility and PA. The detrimental effect of this widespread allele type underscores the opportunity to increase the nutritional value of sorghum grain. Differences caused by the allele types were found to be both heritable and occur regardless of genotypic background. Variations in activity appear to be due to missense mutations that reside in the N-terminal domain of the peptide encoded by the less-common allele type. Although lower in frequency, this allele does not seem to have pleiotropic effects on fitness (for example, yield and plant growth). Selecting for this low-frequency allele in modern breeding programs may result in increased efficiency of energy recovery from cultivated sorghum. Overall, this study clearly demonstrates that naturally occurring allelic variation in starch metabolic genes can increase caloric value without pleiotropic effects. These results underscore the key role that starch-biosynthesis genes, which are conserved across all cereals, can have in addressing food security while minimizing agricultural expansion [3] , [21] . Identification of non-synonymous mutations in pullulanase S orghum b icolor PUL LULANASE ( SbPUL , Sb06g001540 ) is annotated in the v1.0 proteome as a locus spanning ~14.6 kb exclusive of 5′ and 3′ regulatory regions [22] . Pullulanase exists as a single copy in the sorghum genome. No other starch metabolic genes were observed in the annotations of loci within 1 Mb of the pullulanase locus. We sequenced a 1.3-kb fragment in the 5′ genic region of 143 globally distributed accessions spanning modern breeding programme stock to landraces from traditional cropping systems. In silico analysis for missense mutations revealed polymorphisms, leading to two coinciding non-conservative amino-acid changes that depart from the peptide arising from the predicted Sb06g001540.1 gene model ( www.phytozome.com ) [22] . The polymorphisms encode G32R and D105A amino-acid changes that both reside in the N-terminal domain ( Fig. 1 ). Furthermore, we identified the presence of a 24-bp deletion that occurs in all haplotypes carrying Arg and Ala residues at positions 32 and 105, respectively. Together these polymorphisms define the SbPUL-RA allele type. The SbPUL-GD allele type, in contrast to SbPUL-RA , does not possess the 24-bp deletion and encodes Gly and Asp residues at positions 32 and 105, respectively. 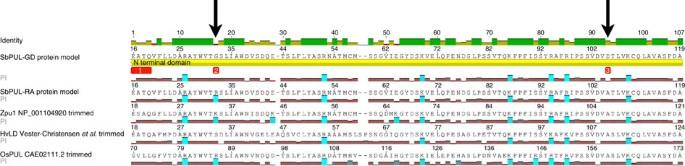Figure 1: Pile-up diagram of cereal pullulanase peptide sequences of the N-terminal domain region. Black arrows highlight variant amino-acid positions between sorghum pullulanase allele types. Amino-acid tracks are given with pI tracks below; pI track bars are proportional to residue charge (positive is tall and blue; negative is low and black). From top to bottom the sequence tracks are: graphical representation of level of consensus identity, SbPUL-GD region with four amino acids found to differ fromSb06g001540.1gene model (red underlay labelled 1) and the two polymorphic residues responsible for the GD to RA transition (red underlay labelled 2 and 3), SbPUL-RA, Zpu1 fromZea mays(NP_001104920), HvLD fromH. vulgare(after Vester-Christensenet al.25), and OsPUL fromOryza sativa(CAE02111.2). Figure 1: Pile-up diagram of cereal pullulanase peptide sequences of the N-terminal domain region. Black arrows highlight variant amino-acid positions between sorghum pullulanase allele types. Amino-acid tracks are given with pI tracks below; pI track bars are proportional to residue charge (positive is tall and blue; negative is low and black). From top to bottom the sequence tracks are: graphical representation of level of consensus identity, SbPUL-GD region with four amino acids found to differ from Sb06g001540.1 gene model (red underlay labelled 1) and the two polymorphic residues responsible for the GD to RA transition (red underlay labelled 2 and 3), SbPUL-RA, Zpu1 from Zea mays (NP_001104920), HvLD from H. vulgare (after Vester-Christensen et al . [25] ), and OsPUL from Oryza sativa (CAE02111.2). Full size image Comparisons of SbPUL against available sequences cDNA sequence from SbPUL-GD grain was used to validate the incorporation of these variant codons in Sb06g001540 transcripts and to test the structure of the Sb06g001540.1 gene model. The cDNA sequence confirmed incorporation of the polymorphisms described above. First, we noted errors in the splice boundaries annotated for the Sb06g001540.1 5′ region, including the addition of 12 bp to the end of exon 1 and the omission of exon 2 altogether. The differences in exon structure changed the sequence of the predicted SbPUL-GD peptide into closer agreement with pullulanases from other cereals. However, SbPUL-GD differs significantly from barley, maize and rice at positions 32 and 105. Peptide sequences from loci, most homologous to Sb06g001540.1 in maize, rice and barley, highlight the deviations from these cereal pullulanases that the SbPUL-GD N-terminal sequence exhibits in MUSCLE alignments ( Fig. 1 ) [23] . Polymorphic residues 32 and 105 in sorghum both occur in conserved islands of sequence among the cereals, but with residues 32 and 33 in barley being swapped in position relative to homologous positions in other cereals. More importantly, we found that the SbPUL-RA form shares greater similarity at the amino-acid level to maize, rice and barley at residue 32/33 and is identical to other cereal pullulanases at residue 105 in comparison with SbPUL-GD. To further test the distinct nature of SbPUL-RA allele types, we assembled a gene tree from 42 resequenced lines and found that SbPUL-RA alleles diverge dramatically from SbPUL-GD ( Fig. 2 ). Superimposing our sorghum gene models onto the Hordeum vulgare limit dextrinase (HvLD) three-dimensional structure revealed that these residues are solvent exposed and proximal to one another in the folded peptide ( Supplementary Fig. S1 ) [24] , [25] . This implies that the SbPUL-RA allele product resembles other cereal pullulanases in these conserved regions both in primary sequence and possibly in peptide chemical properties within the region. These residues are exposed to the extra-molecular environment, increasing the likelihood of inter-molecular or functional significance for these polymorphisms. It has been proposed that the N-terminal domain, although poorly defined functionally, forms one-half of a pore, leading to the catalytic region in HvLD. In vivo support for this function, however, is lacking at present in cereals [25] . Identification of the variant SbPUL-GD allele type will allow further biochemical studies of sorghum pullulanase and may shed insight into the function of the N-terminal domain. 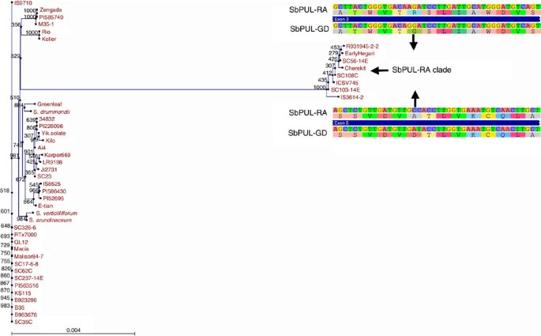Figure 2: Gene tree displaying the well-defined clade of SbPUL-RA allele types. Gene tree ofSbPULsequences spanning the genomic sequence from the predicted start and stop ofSb06g001540.1. Insert windows in the upper right depict the polymorphisms of interest in exon 3 and exon 5. Figure 2: Gene tree displaying the well-defined clade of SbPUL-RA allele types. Gene tree of SbPUL sequences spanning the genomic sequence from the predicted start and stop of Sb06g001540.1 . Insert windows in the upper right depict the polymorphisms of interest in exon 3 and exon 5. Full size image SbPUL-RA confers increased digestibility in isogenic lines To test whether SbPUL-GD and SbPUL-RA allele types differ in their PA and digestibility in a genetically homogenous background, we generated a F 6 near-isogenic line (NIL) by single-seed decent by selecting seeds from a heterozygous individual arising in each generation. Grain obtained from segregating genotypes was tested through four generations (F 3 , F 4 , F 5 and F 6 ) for PA using an assay that measures α 1→6 bond cleavage between maltriose subunits of the polysaccharide substrate. Overall, we found that SbPUL-RA grain possessed significantly higher PA than SbPUL-GD (analysis of variance (ANOVA): df=31, F RA−GD =17.62, P RA−GD =0.0002; see Fig. 3a and Supplementary Table S1 ). In fact, the PA of SbPUL-RA was found to be 67% greater than that of SbPUL-GD . Heterozygous grain, on the other hand, was statistically indistinguishable from SbPUL-GD and SbPUL-RA , (ANOVA: df=31; F RA−HET =2.62, P RA−HET =0.115; F GD−HET =2.77, P GD−HET =0.106; see Fig. 3a and Supplementary Table S1 ). Heterozygote PA values were between that of the homozygotes. The lack of significant difference between heterozygotes and homozygotes is probably because of the greater amount of variability in heterozygous lines. Taken together, the polymorphisms described above, the lack of any nearby annotated gene that may have an effect, and the pullulanase enzyme assay, all strongly support our hypothesis that SbPUL allele type underlies the effects described here. 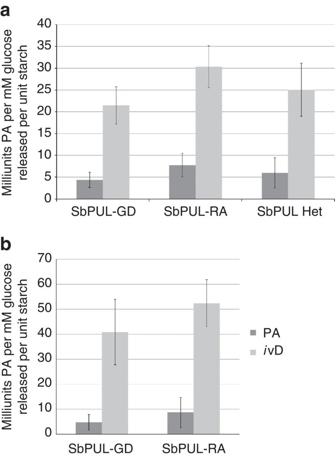Figure 3: Comparison of PA andivD of the NIL and diverse genotype sets. (a) PA (n=8 of each genotype with two technical replicates) andivD (n=3 of each genotype with two technical replicates) of NILs homozygous for either theSbPUL-GDorSbPUL-RAallele, or heterozygous at theSbPULlocus. (b) PA andivD of dNIRS genotype set (n=36). For both figure panels y-axis units are miliunits of α 1→6 glucosidic bond cleavage activity and glucose released (unit total starch)−1for PA andivD, respectively. Dark grey and light grey bars are PA andivD values, respectively. Error bars represent 1 s.d. from the mean. Figure 3: Comparison of PA and iv D of the NIL and diverse genotype sets. ( a ) PA ( n =8 of each genotype with two technical replicates) and iv D ( n =3 of each genotype with two technical replicates) of NILs homozygous for either the SbPUL-GD or SbPUL-RA allele, or heterozygous at the SbPUL locus. ( b ) PA and iv D of dNIRS genotype set ( n =36). For both figure panels y-axis units are miliunits of α 1→6 glucosidic bond cleavage activity and glucose released (unit total starch) −1 for PA and iv D, respectively. Dark grey and light grey bars are PA and iv D values, respectively. Error bars represent 1 s.d. from the mean. Full size image Using the F 6 NILs, we then tested whether the pullulanase allele types would show differences in their digestibility. This was done using an in iv D assay that was designed as a proxy of the monogastric digestive system using porcine digestive enzymes [26] . Overall, we found that the SbPUL-RA grain showed significantly higher iv D than both the SbPUL-GD and heterozygote grain (ANOVA: df=5; F RA−GD =14.68, P RA−GD =0.018; F RA−HET =11.13, P RA−HET =0.028; F GD−HET =2.72, P GD−HET =0.174; see Fig. 3a and Supplementary Table S2 ). On average, we found that the iv D of the SbPUL-RA grain was 41% higher than that of the SbPUL-GD grain and 21% higher than that of the SbPUL heterozygote grain. The SbPUL-RA phenotype is expressed irrespective of genotype To ensure the reliability of the observed differences in PA and iv D between the two pullulanase allele types isolated in the NIL, we replicated the PA and iv D analyses using a panel of 36 accessions. These were selected on their diverse near-infrared spectra (dNIRS) of grain representing elite hybrid parents and landraces used in the Queensland sorghum breeding programme. We found that, on average, the genotypes carrying the SbPUL-RA allele type had significantly higher iv D than the genotypes carrying the SbPUL-GD allele type (general linear mixed model (GLMM) fitted with a binomial distribution and genotypes as random effects: PUL allele~ iv D; df=34; estimate=0.35; s.e.=0.11; t =3.04; P =0.0045; see Fig. 3b and Supplementary Table S3 ). The average iv D of the genotypes carrying the SbPUL-RA allele type was 28% higher than the genotypes carrying the SbPUL-GD allele type. In contrast to the NIL, we did not find that genotypes carrying the SbPUL-RA allele type had significantly higher PA than the genotypes carrying the SbPUL-GD allele type (GLMM fitted with a binomial distribution and genotypes as random effects: PUL allele~PA; df=34; estimate=0.24; s.e.=0.13; t =1.83; P =0.075; see Fig. 3b and Supplementary Table S3 ). The average PA of the genotypes carrying the SbPUL-RA allele type was, however, 82% higher than the genotypes carrying the SbPUL-GD allele type. Furthermore, we did find that PA was significantly positively correlated with iv D (LMM with genotypes as random effects: PA~ iv D; df=34; estimate=0.156; s.e.=0.047; F=10.76; P =0.0024). This suggests that, in comparison with iv D, PA had greater sensitivity to the wide genetic and developmental variability of the accessions included in the dNIRS set. Overall, our results demonstrate that sorghum accessions homozygous for the SbPUL-RA allele showed higher iv D than sorghum accessions carrying the SbPUL-GD allele, regardless of the genetic background. SbPUL-RA occurs at a reduced frequency Given the apparent advantage that the SbPUL-RA allele type has upon digestibility, it seems intuitive that such a beneficial allele type would be in the majority of cultivated sorghum. Surprisingly, we did not find this to be the case. In addition to sequencing 149 lines mentioned above, we genotyped 70 lines using primers amplifying across the associated 24-bp deletion in SbPUL-RA , for a total of 219 globally distributed genotypes from modern breeding programs and landraces. Indeed, the SbPUL-RA allele type occurs at a low frequency, five times less than the frequency of SbPUL-GD (SbPUL-RA=15.07%, SbPUL-GD=82.65%, het=2.28%; Supplementary Table S4 ). This strongly highlights the potential that increasing the frequency of SbPUL-RA may provide a way to improve the nutritional value of sorghum. No deleterious effects are associated with SbPUL-RA Within the Queensland sorghum breeding programme, a yield trial of BC 2 F 1 hybrids in a well-adapted genetic background allowed us to compare the mean yield of heterozygotes with that of SbPUL-GD homozygotes. We found that the mean yield of heterozygous hybrids (5.44 t/ha, n =94) was not significantly different from the mean yield of homozygous SbPUL-GD hybrids (5.37 t/ha, n =82). In fact, the frequency of SbPUL-RA homozygotes in accessions taken from the Queensland breeding programme is 21.43%, a rate that is higher than other genotype panels examined that furthermore suggests no deleterious effect ( Supplementary Table S4 ). There was also no support for deleterious differences between our NIL homozygous for either allele type. Plant phenology of our F 6 NILs grown in a field setting showed no effects that would impinge on the viability of SbPUL-RA within modern agriculture. NIL genotypes exhibited a narrow range of variability. SbPUL-RA plants took an additional 3.6 days to flower on average while producing ~0.78 more leaves than SbPUL-GD plants ( Supplementary Table S5 ). The underlying cause of these differences may be because of linkage drag of known maturity loci on SBI-06. Taken together with the Queensland breeding programme data, the NIL data demonstrate that the increased digestibility conveyed by the SbPUL-RA allele type are not offset by negative pleiotropic effects on plant growth and yield. Sorghum is drought stress tolerant, and because of that attribute, there has been much interest in it as a crop that will ensure food security, particularly in places negatively affected by climate change such as sub-Saharan Africa [5] , [7] . About 50% of the calories consumed by the world’s poor are from maize, rice and wheat, whereas these cereals provide only 31% of the calories consumed in sub-Saharan Africa [5] . The digestibility of sorghum grain, however, is lower per unit mass than maize, despite containing starch at similar levels to other major grains [8] . In this paper, we have demonstrated that a low-frequency allele type of the pullulanase locus increases digestibility without tradeoffs in the form of negative pleiotropic effects, thus adding value to a crop pre-adapted to drought and heat stress. Improvement to the digestibility and caloric value of sorghum has been sought for decades, but most mutations that increase digestibility of this crop have been met with tradeoffs in other agronomic traits. For example, previous attempts to introduce sorghum expressing the waxy phenotype, leading to increased nutritive value, failed primarily because the yield of waxy varieties was significantly reduced [27] . Similarly, tannin content of sorghum negatively affects its value as a food source and it is possible to breed for low tannin grain, but low tannin varieties with higher digestibility are prone to bird damage in the field [20] . In contrast to the studies above, we found no evidence that the SbPUL-RA allele type has a negative effect on yield or a deleterious effect on field grown plants in Australian breeding trial data and our F 6 NILs, respectively. The amino acids at positions 32 and 105 in the predicted SbPUL-RA peptide are identical or more similar to other cereal pullulanases, and, thus, it is reasonable to say that SbPUL-RA polymorphisms are more akin to a restoration of function from the loss-of-function that the SbPUL-GD allele type displays. Because of this hypothetical restoration of function, by conversion of the pullulanase allele type at this locus, it is unsurprising that no detrimental effects on yield are observed. Further research should now focus on to quantifying the gains in agronomic systems and nutrition possible through in vivo digestibility experiments. An additional avenue of enquiry focuses upon the specific biochemical properties of purified SbPUL isoforms and their expression levels in vivo to fully characterize the basis of the effect we describe. We speculate that the utilization of directed breeding to introgress the SbPUL-RA allele type into elite varieties of cultivated sorghum can help improve the caloric value of this staple food. Ultimately, increasing the caloric value of this crop without reducing yield can help to ensure global food security in drought-prone areas of Africa, Asia and elsewhere, while minimizing negative effects of agricultural expansion. Plant material A diverse panel of 240 genotypes was screened by NIRS at the Queensland Government Leslie Research Centre (Toowoomba, Queensland, Australia). The panel consisted of genotypes from the United States, Oceania, Asia and Africa, with representatives from modern and traditional breeding origins. Of these, a subset were selected based on having the most divergent spectra. An unreleased F 1 hybrid (hybrid: A1*9_B004216/R002133 ), produced by the Department of Agriculture, Fisheries and Forestry, Queensland, was found to be heterozygous at Sb06g001540 by Sanger sequencing. F 2 plants were genotyped as detailed below before obtaining the F 3 grain used for subsequent analysis. Similarly, F 3 plants were genotyped and F 4 grain was used for subsequent analysis, and so forth till the F 6 generation. In each generation, the population consisted of plants obtained through single-seed descent from a chosen heterozygous individual, and all heads were bagged before anthesis to prevent contamination of developing segregating heads. Genotyping and sequencing of gene fragments Plant leaf samples were collected fresh or stored dried and extracted with a CTAB buffer method as described by Laidlaw et al . [28] . PCR for genotyping was carried out with Bioline MyTaq HS ( www.bioline.com.au ) per the manufacturer’s protocol. To obtain amplicons that were sequenced, we used primers developed by Hamblin et al . : Pul1-F1 5′-GTTGCGGAGTATTATCGCTTGG-3′ and Pul1-R1 5′-AGGCTCAAAGGCTTCTAAAATCG-3′ [27] . To genotype dNIRS and Landrace panel accessions possessing either SbPUL-RA or SbPUL-GD type alleles, we sequenced the 1.37-kb PCR product by Sanger sequencing followed by data analysis in Geneious ( www.biomatters.com ). Sequences for the dNIRS were previously released [29] . Sequences for the Landrace set where the genotype was homozygous are available in GenBank ( www.ncbi.nlm.nih.gov/genbank/ ) in 91 sequential accessions between accession numbers KC338900 and KC338990 . For rapid screening, we designed and utilized a primer pair amplifying a genomic fragment spanning a 24-bp deletion present in SbPUL-RA allele types. The resulting SbPUL-GD and SbPUL-RA amplicons are 404 and 380 bp in length, respectively. Primer sequences for the size marker PCR are: PULmark-F 5′-TCACACGAACGCCATCCACC-3′ and PULmark-R 5′-TAGTGGGGCAATGAACCATCCAAGG-3′. Scoring was performed by visualization of size differences using a standard 1 × Tris-borate buffer and 2% agarose gels and compared with controls of known genotype by Sanger sequencing. Protein sequence alignment and three-dimensional modelling The predicted peptide sequence was based on Sb06g001540.1 in the Sbi1.4 gene set as retrieved from Phytozome ( www.phytozome.com ) based on the available whole-genome sequence and annotated by various means [22] . The most homologus BLASTP hits for maize, rice and barley were retrieved and compared by MUSCLE alignment in Geneious ( www.biomatters.com ). The predicted SbPUL peptide sequence was manipulated to mark non-silent polymorphisms and trimmed to match the starting methionine determined by comparison with other cereal sequences in MUSCLE alignments. The Phyre server ( www.phyre.com ) was queried with the predicted SbPUL-RA peptide sequence [24] . Analogous positions for SbPUL residues 32 and 105 on the HvLD structure (ProDB no. 2Y4S) were highlighted in Protein Data Bank ( www.rcsb.org/pdb ) Protein Workshop software. iv D measurements iv D was calculated for each line of the dNIRS set by finding the quotient of glucose released after 4 h of artificial digestion over total starch content. The iv D methodology is detailed in Sopade and Gidley [26] , but the following is a brief overview. All grain was ground using a TEFAL Prep Line 650 coffee grinder ( www.tefal.com.au ) until a uniform fine powder was obtained for all samples. Total starch content was measured using 50 mg of ground grain with the Megazyme Total Starch Assay ( www.megazyme.com , product code K-TSTA). A total of 500 mg of ground grain was used to measure in vitro starch digestibility. The quotient of in vitro starch digestibility over total starch content is therefore a proportional figure and independent of starch content in diverse genotypes. Pullulanase/limit dextrinase assays Limit dextrinase assays using pullulan–azurine ( www.megazyme.com , product code T-LDZ200) as a substrate were performed on sorghum grain samples ground with a mortar and pestle for 3 min or until uniform fine particles were obtained. Samples were processed from that point onward as described by the Megazyme Limit Dextrizyme kit protocol, except the 25 mM dithiothreitol was replaced with 50 mM β-mercaptoethanol in the sodium maleate buffer of the protocol to recapitulate the molar equivalent of reducing power. Field trial for NILs The F 6 population ( n =191) was sown at the University of Queensland, Gatton Campus, on deep, medium-clay, alluvial soil into a 5 × 5 m area. Plots consisting of either homozygote line or segregating plants arising from a heterozygous parent were randomized among 10 rows of 2.5 m each. The experiment contained three replications for SbPUL-GD and SbPUL -heterozygotes and four replications for SbPUL-RA . Five weeks after planting, 6 kg of sulphur-coated urea was applied to enhance plant development. Plants were watered as needed with the irrigation water providing for potassium nutrition. Measurements were taken twice per week and included plant height from soil surface to top leaf attachment and the number of fully expanded leaves. Inflorescences were bagged upon emergence to prevent outcrossing. Days to flowering were recorded for each plant as the number of days between planting and when ~50% of the florets in an inflorescence reached anthesis. Analysis of yield effects in the Queensland breeding programme The BC 2 F 1 yield trial was established to compare a suite of hybrids developed by selecting a large set of BC 1 F 4 lines for superior yield then back-crossing to the recurrent parent once more. The trial had a partially replicated design and was sown, grown, harvested and analysed according to standard breeding programme best practice. The donor parents of these lines were screened with Sb06g001540 allele-specific markers. Then whole-genome marker profiles were used to impute the Sb06g001540 alleles of the BC 2 F 1 hybrids. Only hybrids that could be unambiguously assigned to a pullulanase allele class (either homozygous SbPUL-GD or heterozygous SbPUL-GD/SbPUL-RA ) were included in the yield comparison. The homozygous SbPUL-GD class included 82 hybrids derived from 42 donor parents. The heterozygous SbPUL-GD/SbPUL-RA class included 94 hybrids derived from 40 donor parents. Then a simple one-tailed t -test was used to compare the hybrids in these two classes. Statistical analyses ANOVA values were calculated using the PopTools package ( www.poptools.org ). GLMM analyses were performed using the R statistical package MASS [30] . LMM analyses were performed using the R statistical package nlme [31] . Gene tree A gene tree was constructed using CLC Genomics Workbench software ( www.clcbio.com ) from a total of 45 resequenced sorghum lines. Three of the lines have been reported previously by Zheng et al . [32] The remaining 42 lines have been resequenced as part of a consortium between the Department of Agriculture, Forestry and Fisheries, Queensland, the University of Queensland and Beijing Genome Institute. Accession codes: The sequences for the Landrace set where the genotype was homozygous have been deposited in GenBank under accession codes KC338900 to KC338990 . How to cite this article: Gilding, E. K. et al . Allelic variation at a single gene increases food value in a drought-tolerant staple cereal. Nat. Commun. 4:1483 doi: 10.1038/ncomms2450 (2013).